Fast vacancy-mediated oxygen ion incorporation across the ceria–gas electrochemical interface Electrochemical incorporation reactions are ubiquitous in energy storage and conversion devices based on mixed ionic and electronic conductors, such as lithium-ion batteries, solid-oxide fuel cells and water-splitting membranes. The two-way traffic of ions and electrons across the electrochemical interface, coupled with the bulk transport of mass and charge, has been challenging to understand. Here we report an investigation of the oxygen-ion incorporation pathway in CeO 2-δ (ceria), one of the most recognized oxygen-deficient compounds, during hydrogen oxidation and water splitting. We probe the response of surface oxygen vacancies, electrons and adsorbates to the electrochemical polarization at the ceria–gas interface. We show that surface oxygen-ion transfer, mediated by oxygen vacancies, is fast. Furthermore, we infer that the electron transfer between cerium cations and hydroxyl ions is the rate-determining step. Our in operando observations reveal the precise roles of surface oxygen vacancy and electron defects in determining the rate of surface incorporation reactions. Electrochemical reactions taking place at the interface between a metal or semiconductor electrode and an electrolyte have been investigated extensively and are relatively well understood [1] , [2] . At these interfaces, electrons are transferred between the solid and redox species in solution, and can be described by formalisms developed originally by Butler and Volmer [2] and Marcus [3] . However, electrochemical reactions in many technologically relevant systems, such as batteries and fuel cells, involve not only the electron transfer process mentioned above, but also the simultaneous incorporation of ions into the electrodes ( Fig. 1 ). Examples include the co-transfer of lithium ions and electrons in mixed ionic and electronic conductors (MIECs) for battery electrodes [4] , and the co-transfer of oxygen ions and electrons in MIECs for solid-oxide fuel cell electrodes [5] . Examples of non-electrochemical incorporation reactions include metal-oxide thermochemical water splitting [6] and oxygen storage in emission control catalysts [7] . However, despite the technological importance of the ion incorporation reactions, they are not well understood. The electrochemical double layer at the solid–liquid or solid–gas interfaces is complex, and involves the interactions of mobile ions and electrons in the solid state, adsorbates and electrostatic fields [8] , [9] . A complete understanding of ion incorporation reactions at the surface of MIECs could lead to the development of new materials with facile reactivity for applications in energy conversion/storage and chemical transformations. 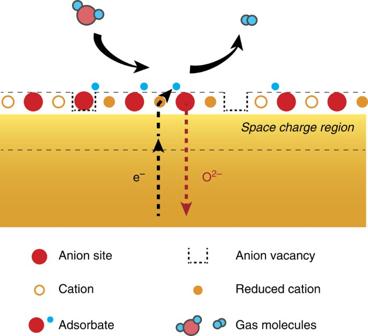Figure 1: Schematic illustration of the oxygen-ion incorporation pathway. The incorporation process at the surface of mixed ionic-electronic conductors consists of the adsorption/desorption of gas molecules, the dissociation/association/diffusion of adsorbates, the transfer of electrons and ions across the interface, and the transport of electrons and ions between the surface and the bulk. Figure 1: Schematic illustration of the oxygen-ion incorporation pathway. The incorporation process at the surface of mixed ionic-electronic conductors consists of the adsorption/desorption of gas molecules, the dissociation/association/diffusion of adsorbates, the transfer of electrons and ions across the interface, and the transport of electrons and ions between the surface and the bulk. Full size image One of the most studied materials for oxygen-ion incorporation is cerium oxide or ceria [10] , [11] , [12] , [13] , [14] , [15] . Ion-incorporation reactions at the ceria–gas interface are coupled to a wide range of molecules including H 2 /H 2 O, CO/CO 2 , NO x , SO x , etc [10] . Recently, doped ceria was found to exhibit remarkable activity towards hydrogen oxidation and water splitting reactions (HOR and WSR, respectively), which exceeds that of precious metal catalysts. Thus, ceria is becoming a gold standard system to gain insights into designing electrochemically active compounds [16] , [17] . The WSR, typically taking place at temperatures between 400 and 700 °C, is written as: where denotes an oxygen vacancy, denotes an oxygen ion and denotes a Ce 3+ localized electron or a small polaron, using the Kröger–Vink notation. The electrochemical incorporation process comprises a series of steps: adsorption of gas molecules onto the oxide surface, ion/electron transfer across the interface and ion/electron migration from the surface to the bulk ( Fig. 1 ). The surface of ceria has been studied extensively [5] , [18] , [19] . The majority of these work considered the surface and intermediate species at equilibrium. For example, density functional calculations predicted reduced defect formation energy on the low-index surfaces of ceria from that of the bulk [20] , [21] , [22] , [23] , which has been validated experimentally [24] . In operando techniques such as in-situ X-ray photoelectron spectroscopy (XPS) [25] , [26] , [27] , [28] , [29] have also been applied to ceria [16] , [30] , [31] , [32] . However, many of these experiments adopted electrochemical cell geometries that are bulk-diffusion-limited, rather than surface-reaction-limited. As such, these experiments reveal the bulk-like diffusion of oxygen ions and polarons instead of the surface incorporation reaction. It is also worth noting that virtually all spectroscopic work infers the oxygen vacancy concentration from the Ce 3+ concentration using the electroneutrality approximation, which usually breaks down near interfaces. Importantly, this approximation leaves oxygen vacancies, the primary species in the incorporation reaction, out of the picture. Thus, despite recent progress, the oxygen-ion incorporation pathway in ceria remains elusive. In this work, we investigate the oxygen-ion incorporation pathway in ceria during WSR and HOR. We fabricate a model electrochemical cell with thin-film samarium-doped ceria (SDC) as the working electrode and yttria-stabilized zirconia (YSZ) as the solid electrolyte. By adopting a surface-reaction-limited electrochemical cell, we control the overpotential across the solid–gas electrochemical double-layer precisely. Using synchrotron-based ambient pressure XPS (APXPS), we probe the dynamics of surface oxygen, electrons and adsorbates at the solid–gas interface for a wide range of overpotentials. We show that HOR and WSR on ceria proceed via intermediates (hydroxyl ions incorporated on surface oxygen vacancies). The rate of the H 2 O interaction with surface oxygen vacancy is fast, resulting in the total saturation of surface oxygen vacancies with hydroxyl ions under both WSR and HOR conditions. Furthermore, enabled by the rapid transport of oxygen vacancy and localized electron between the bulk and the surface, the surface is persistently enriched with these key reactants during the HOR and WSR by up to four orders of magnitude over bulk concentrations. The abundance, high reactivity and fast transport of these defects at large overpotentials are crucial for catalysing the incorporation reactions. These in operando observations reveal the precise roles of oxygen vacancy and electron defects in promoting the rate of surface incorporation reactions in ceria, and suggest the origin of the high electro-catalytic activity. Electrochemical characteristics The solid-state electrochemical cell was characterized in 260 mTorr of H 2 /H 2 O/Ar atmosphere at 500 °C ( Fig. 2a ). These conditions approach those of technologically relevant solid-oxide fuel cells, electrolyzers and water-splitting membranes. The Sm-doped CeO 2 thin film exhibits mixed ionic and electronic conductivity, with a bulk ionic conductivity of ~7 mS cm −1 and an electronic conductivity of ~6 mS cm −1 at open-circuit conditions [33] (see Supplementary Methods ). Under cathodic bias (WSR, the forward direction of equation (1)), oxygen vacancies generated at the counter electrode and electrons from the embedded current collector migrate to the ceria surface and react with the water vapour to generate hydrogen ( Fig. 2a ). Under anodic bias (HOR), the reverse takes place. As these reactions proceed under electrochemical polarization, we used core-level and valence-band photoelectron spectroscopy to probe the steady-state concentrations of oxygen, electron and reaction intermediates on the ceria surface. 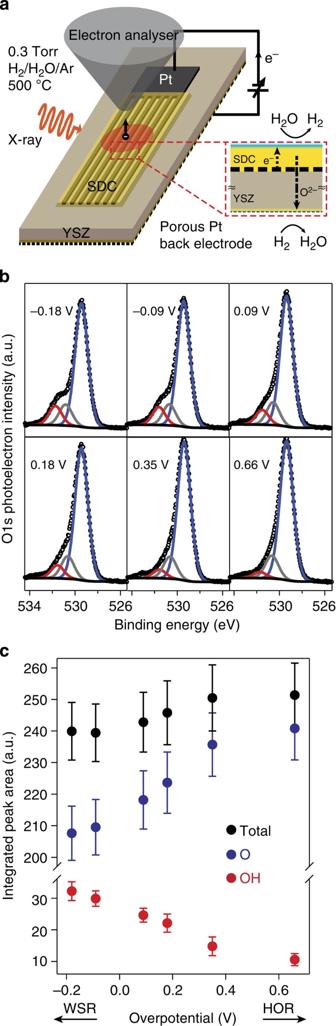Figure 2: Evolution of oxygen species in the electrochemical double-layer with overpotential. (a) A schematic depicting the experimental setup. The cell is based on yttria-stabilized zirconia (YSZ) solid-oxide electrolyte, with dense Sm-doped ceria (SDC) as the working electrode and SDC/porous Pt as the counter electrode. Patterned Pt is embedded in SDC thin film for efficient current collection. (b) Normalized O 1s spectra at 500 °C in 0.3 Torr H2/H2O/Ar. Taken at a photon energy of 690 eV and an probing depth of 0.6 nm. Three components are fitted by constraining equal full-width half-maximum. The main peak in blue and shoulder peaks in grey and red are due to lattice oxygen (O), oxygen bonded to the Si impurity and surface, respectively. The binding energy (BE) is calibrated with the Au 4f7/2peak and the lattice oxygen peaks are aligned at 529.4 eV (BE at open-circuit condition) for easier comparison of peak shapes. The intensity is normalized to the pre-edge background. (c) The normalized peak areas of lattice O and adsorbedas a function of overpotential. The error bars account for the fluctuation in the pre-edge background intensity as well as peak fitting uncertainties. Figure 2: Evolution of oxygen species in the electrochemical double-layer with overpotential. ( a ) A schematic depicting the experimental setup. The cell is based on yttria-stabilized zirconia (YSZ) solid-oxide electrolyte, with dense Sm-doped ceria (SDC) as the working electrode and SDC/porous Pt as the counter electrode. Patterned Pt is embedded in SDC thin film for efficient current collection. ( b ) Normalized O 1s spectra at 500 °C in 0.3 Torr H 2 /H 2 O/Ar. Taken at a photon energy of 690 eV and an probing depth of 0.6 nm. Three components are fitted by constraining equal full-width half-maximum. The main peak in blue and shoulder peaks in grey and red are due to lattice oxygen (O), oxygen bonded to the Si impurity and surface , respectively. The binding energy (BE) is calibrated with the Au 4f 7/2 peak and the lattice oxygen peaks are aligned at 529.4 eV (BE at open-circuit condition) for easier comparison of peak shapes. The intensity is normalized to the pre-edge background. ( c ) The normalized peak areas of lattice O and adsorbed as a function of overpotential. The error bars account for the fluctuation in the pre-edge background intensity as well as peak fitting uncertainties. Full size image Adsorbate–vacancy interaction The O 1s core level spectra vary systematically with the applied overpotential ( Fig. 2b ). We identified a total of three oxygen species at an information depth of ~0.6 nm (for the definition of surface sensitivity see Supplementary Methods ). Based on earlier photoemission studies, we assigned the most intense peak (shown in blue and denoted as O) to the bulk-like lattice oxygen [34] , [35] . A smaller peak ~1.3 eV higher in binding energy (shown in grey and denoted as O') is attributed to oxygen bonded to segregated silicon impurities ( Supplementary Fig. 1 ). This impurity peak, which reaches a maximum atomic fraction of 14% of the oxygen photoelectron spectra, does not change appreciably with bias over the course of the experiment. Finally, the photoelectron peak with the highest binding energy (~2.2 eV higher than the lattice oxygen peak) is assigned to adsorbed OH − groups, consistent with prior photoemission and temperature-programmed desorption investigations [34] , [35] , [36] , [37] . We note, however, the binding energy is considerably larger than that reported by Zhang et al. [32] Moreover, we observed that the binding energy difference between the OH and the lattice O changed with bias ( Supplementary Fig. 2 ). Such a bias-dependent shift was also observed previously by Zhang et al. [32] , and has been attributed to a change in the potential drop across the electrochemical double-layer. However, it is unclear which fraction of the potential drop along the double-layer assists the charge-transfer reaction. Owing to the intentional bulk diffusional polarization in that work, a direct comparison with the present result is not possible. Under nominally dry conditions, the photoelectron peak attributed to OH − disappears entirely, lending another support to our assignment. In principle, the OH − peaks could arise from both OH − groups bonded to Ce atoms or incorporated in surface oxygen vacancies (see Supplementary Fig. 3 ). To quantify the dynamics of oxygen species as a function of overpotential, the oxygen spectra were normalized by the background intensity above the O 1s photoelectron peak. This normalization approach is justified by the negligible change in the cation composition of the sample and, thus, the inelastic contribution to the background photoelectron signal. This normalization procedure was further verified independently by concurrent APXPS measurements of a gold foil Fermi-coupled to the ceria electrode. For details on peak assignment and normalization procedures, see Supplementary Methods . As can be seen in the normalized spectra, the most striking behaviour of surface oxygen species ( Fig. 2b ) is the counter-correlation between the bulk-like lattice oxygen and OH − intensities as a function of overpotential. Although the intensity of the bulk-like oxygen peak decreases under WSR conditions, that of the OH − peak increases, and vice-versa under HOR conditions. This behaviour is shown quantitatively in Fig. 2c . The sum of the bulk-like oxygen and OH − peak area is, within error, invariant with the overpotential. This observation immediately suggests that the surface hydroxyl occupies and saturates the electrochemically generated oxygen vacancy sites on the surface regardless of the reaction rate (that is, the current) for both WSR and HOR. This species is thus denoted as . We note that surface and sub-surface oxygen vacancies cannot be differentiated at an information depth of 0.6 nm (ref. 38 ), and that the physical location of may not coincide exactly with the surface oxygen site [39] . Even in the absence of quantitative analysis, these dynamic observations reveal a crucial feature of the oxygen-ion incorporation pathway. Under WSR conditions, oxygen vacancy migrating from the bulk (driven by the polarization) is immediately refilled by a surface hydroxyl. Under HOR conditions, on the other hand, surface hydroxyl groups are released rapidly when the oxygen vacancies migrate from the surface to the bulk (also driven by the polarization). In other words, the interaction of H 2 O with the surface oxygen vacancies is sufficiently facile that the ion incorporation/removal process is quasi-equilibrated under both WSR and HOR conditions. To the best of our knowledge, this is the first direct experimental evidence showing the fast vacancy-mediated ion incorporation reaction. This observation also agrees with the density-functional theory calculations under equilibrium conditions [35] , [40] , [41] , [42] , [43] , [44] and measurements under static conditions, where water molecules adsorb and dissociate preferentially at the surface oxygen vacancy site in CeO 2−x (ref. 45 ) and in TiO 2−x (ref. 46 ). Migration and segregation of oxygen vacancies Having shown quantitatively that incorporates into surface oxygen vacancies in ceria and that the reaction is fast for the range of overpotentials probed, we now turn to the near-surface transport of oxygen vacancy from the bulk to the surface ( Fig. 2a ). This is another essential step of the ion-incorporation reaction. Under our measurement conditions, Sm-doped ceria exhibits negligible bulk diffusional polarization compared with the magnitude of the applied overpotential (see Supplementary Methods ). Little understood, however, is the bulk-to-surface oxygen transport resistance, which can differ substantially from bulk values because of surface traps and a depletion layer in the space-charge region [5] , [47] , [48] . We examined the possibility that near-surface oxygen ion transport is rate determining by quantifying the oxygen concentration and the electrostatic potential gradients near the surface under reaction conditions. Oxygen vacancy diffusion from the bulk to the surface under WSR conditions requires a concentration gradient in excess of that under the open-circuit condition, and vice versa under HOR conditions. Owing to the lack of lateral resolution in our experiment, we discuss the transport gradient that spans from the electrolyte to the solid–gas interface, which dominates based on the defect migration direction depicted in Fig. 1 . However, we cannot completely rule out the presence of microscopic lateral diffusional gradient, for example, due to the slow diffusion of adsorbate to surface oxygen vacancies. Nevertheless, we expect surface diffusion to be rapid compared with the bulk at the temperature investigated. We obtained the cross-plane excess gradient near the surface by taking the difference between the bulk and the surface oxygen vacancy concentration relative to the value at the open-circuit condition ( Fig. 3a ). Based on previously measured oxygen vacancy concentration in the bulk and similarly deposited thin-film ceria [49] , the intrinsic bulk oxygen vacancy concentration (relative to the total oxygen content) under our experimental conditions ranges from 0.6% (at −0.18 V) to 2 × 10 −4 % (at 0.35 V). These values are significantly lower than the extrinsic oxygen vacancy concentration because of Sm doping (5%). On the other hand, the measured concentration of surface oxygen vacancies (saturated with ) ranges from 6% (at −0.18 V) to 3% (at 0.35 V). By comparing these values to those under the open-circuit condition, we computed the excess diffusional gradient as defined in Fig. 3a . A negative value indicates an excess driving force that facilitates bulk-to-surface diffusion, whereas a positive value indicates the opposite. During WSR, oxygen vacancies migrate from the bulk to the surface. However, the observed non-negative excess diffusional gradient is inconsistent with a diffusion-limited process. This evidence suggests that the near-surface diffusion overpotential is negligible. 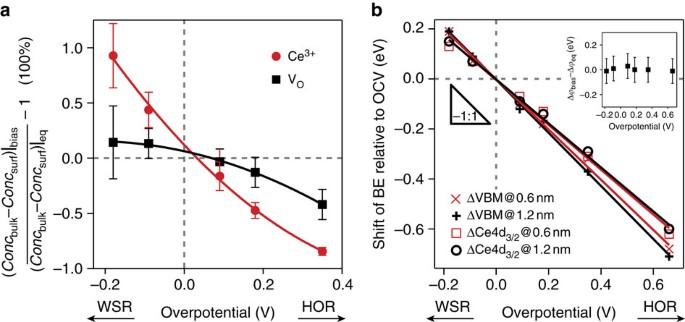Figure 3: The cross-plane transport gradients in the near-surface region. (a) The excess polaron (red circle) and oxygen vacancy (black square) concentration gradients (from bulk to surface) relative to the values at the open-circuit condition. Lines are for guiding the eyes. The error bars account for the uncertainties in both the measurement of surface concentrations and the calculations of bulk concentrations because of fluctuations in the temperature and gas flow ratio. (b) The shifts of valence-band maxima and Ce 4d core level binding energy at two information depths as a function of overpotential. Error bars in the binding energy are about 0.1 eV. Inset: the invariant electrostatic potential in the surface space-charge region upon polarization. Δϕis defined as the difference in the electrostatic potential between a depth of 1.2 and 0.6 nm. Figure 3: The cross-plane transport gradients in the near-surface region. ( a ) The excess polaron (red circle) and oxygen vacancy (black square) concentration gradients (from bulk to surface) relative to the values at the open-circuit condition. Lines are for guiding the eyes. The error bars account for the uncertainties in both the measurement of surface concentrations and the calculations of bulk concentrations because of fluctuations in the temperature and gas flow ratio. ( b ) The shifts of valence-band maxima and Ce 4d core level binding energy at two information depths as a function of overpotential. Error bars in the binding energy are about 0.1 eV. Inset: the invariant electrostatic potential in the surface space-charge region upon polarization. Δ ϕ is defined as the difference in the electrostatic potential between a depth of 1.2 and 0.6 nm. Full size image In addition to the excess oxygen concentration gradient, the excess electrostatic potential gradient in the surface space-charge region was also probed via the rigid shift of photoemission peaks. The binding energy of Ce 4d photoelectron peak at ~123 eV and the valence-band maximum were measured as a function of overpotential at information depths of 0.6 and 1.2 nm ( Fig. 3b ). Given the high doping level and oxygen vacancy concentration, the surface space-charge layer thickness is expected to be on the order of 1–2 nm (ref. 50 ). Thus, our probing depth accesses a significant portion of the space-charge region immediately adjacent to the surface, if present. As shown in Fig. 3b , both the Ce 4d core-level-binding energy as well as the valence-band maximum varied linearly with the Ohmic-corrected overpotential. In fact, the binding energy shifts, referenced to binding energies at the open-circuit condition, are precisely equal to the applied overpotential [25] . This observation confirms that the rate-determining step occurs at the ceria–gas interface, and not in the sub-surface region. Moreover, the rigid shift of both Ce 4d core level peak and valence-band maximum with overpotential at an information depth of 0.6 nm is identical to that of 1.2 nm. Thus, we can conclude that the electrostatic potential between these two depths does not change with electrical current under both WSR and HOR polarizations ( Fig. 3b inset). Combined with the negligible diffusional overpotential upon polarization, this observation confirms that oxygen transport from the bulk to the surface (and vice versa) during incorporation is fast, compared with the rate-determining step. We note that the lack of change in the electrostatic potential profile, despite the significant change in the concentration, could be because of the preservation of charge neutrality (as observed in the bulk of proton-conducting oxides like doped BaZrO 3 (ref. 51 ). It may also relate to the high concentration of near-surface mobile charge carriers available to screen the excess charge. The strong oxygen-ion gradient is understood as non-equilibrium defect segregation, whereby lowered formation energy at the surface relative to that in the bulk leads to enrichment [24] . During incorporation reaction, the persistent segregation of reactive oxygen vacancy from the bulk to the surface arises from the rapid transport of oxygen vacancies under both WSR and HOR conditions. In sharp contrast with transport limitation in surface depletion zone observed in Fe-SrTiO 3 (ref. 47 ), fast oxygen vacancy transport from the bulk to the surface in ceria observed here further assures the availability of oxygen vacancy to participate in the surface electrochemical reaction [38] . The so-called quasi-equilibrium segregation extent of 1 × 10 at −0.18 V (WSR), defined as the ratio of surface to bulk concentration of intrinsic oxygen vacancies, represents significantly enhanced availability of adsorption sites for gas-phase water molecules. Likewise, a dramatic segregation extent of 1 × 10 4 at 0.35 V (HOR) increases the concentration of species that subsequently combine to form H 2 O. Migration and segregation of small polarons In addition to oxygen-containing species, mobile electrons at the surface are also crucial intermediate species that participate in the incorporation reaction by reducing or oxidizing the adsorbed . When Ce is reduced from the 4+ to the 3+ oxidation state, a small polaron (localized electron) occupies the narrow Ce 4f electronic state in the band gap [52] , [53] , [54] . We probed the occupation of the Ce 4f state using both valence-band and core-level photoelectron spectroscopy. 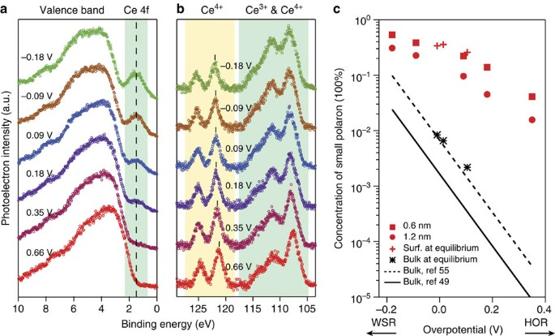Figure 4: Evolution of polaronic electrons with overpotential. (a) Valence-band spectra measured at 500 °C in 0.3 Torr H2/H2O/Ar using a 250-eV photon energy. Information depth is ~0.6 nm. The Ce 4f peak (labelled) directly corresponds to the Ce3+concentration because of normalization by the total Ce intensity. (b) Ce 4d core level spectra measured using a 370-eV photon energy at the same information depth. Spectra are normalized by the total intensity of the Ce 4d peaks. Position of the marked peak is plotted inFig. 3b. (c) Small polaron concentration determined by APXPS at 0.6 and 1.2 nm. Also shown is the surface (+) and bulk (*) polaron concentration under equilibrium conditions, attained by varying the oxygen partial pressure at 521 °C (ref.24). The bulk polaron concentrations are calculated using the reduction energetics data obtained from a similarly prepared Sm0.15Ce0.85O1.925-δthin film (solid line) and a bulk Sm0.2Ce0.8O1.9-δsample (dashed line). Figure 4a,b shows the spectra of valence band and Ce 4d core level normalized to the total Ce 4d intensity (arising from all Ce species). Using two quantification approaches reported previously [24] , [31] , we determined the surface polaron concentration using the Ce 4f intensity as well as the Ce 4d multiplet splitting. Excellent linear correlation was obtained between the two methods ( Supplementary Fig. 4 ), confirming the validity of our quantification approach. Figure 4c shows the concentration of small polarons at an information depth of 0.6 and 1.2 nm under both HOR and WSR conditions. Also plotted is the bulk polaron concentration calculated using the reduction energetics data obtained from a similarly prepared Sm 0.15 Ce 0.85 O 1.925-δ thin film [49] (solid line) and a bulk Sm 0.2 Ce 0.8 O 1.9-δ sample [55] (dashed line). Although the values are slightly different, the calculated surface to bulk concentration ratio is not sensitive to this minor variation in the bulk Ce 3+ concentration. Analogous to the intrinsic oxygen vacancies, the persistent segregation of polarons from the bulk to the surface under electrochemical polarization is dramatic, reaching a segregation extent of more than 2 × 10 at −0.18 V (WSR) and 5 × 10 3 at 0.35 V (HOR) for the surface concentrations quantified at 0.6 nm. As expected, polaron concentration at 1.2 nm is correspondingly lower, but still substantially higher than the bulk values ( Supplementary Fig. 5 ). Another unusual observation is that the oxygen-vacancy-free surface remains mostly in the reduced state, especially under WSR conditions. This stands in contrast to the prevailing view that each oxygen vacancy is charge compensated by two Ce 3+ defects. It appears that the saturating the oxygen vacancies is effectively a positively charged defect, which is then charge compensated by Ce 3+ , similar to the bulk of proton-conducting oxides [51] . Figure 4: Evolution of polaronic electrons with overpotential. ( a ) Valence-band spectra measured at 500 °C in 0.3 Torr H 2 /H 2 O/Ar using a 250-eV photon energy. Information depth is ~0.6 nm. The Ce 4f peak (labelled) directly corresponds to the Ce 3+ concentration because of normalization by the total Ce intensity. ( b ) Ce 4d core level spectra measured using a 370-eV photon energy at the same information depth. Spectra are normalized by the total intensity of the Ce 4d peaks. Position of the marked peak is plotted in Fig. 3b . ( c ) Small polaron concentration determined by APXPS at 0.6 and 1.2 nm. Also shown is the surface (+) and bulk (*) polaron concentration under equilibrium conditions, attained by varying the oxygen partial pressure at 521 °C (ref. 24 ). The bulk polaron concentrations are calculated using the reduction energetics data obtained from a similarly prepared Sm 0.15 Ce 0.85 O 1.925-δ thin film (solid line) and a bulk Sm 0.2 Ce 0.8 O 1.9-δ sample (dashed line). Full size image Next, we turn to the rate at which small polarons migrate from the bulk to the surface during WSR, and vice versa during HOR. We again calculated the cross-plane, excess concentration gradient near the surface. During WSR, we observed a positive excess diffusional gradient for the small polarons ( Fig. 3a ), similar to that for the oxygen vacancies. The sign of the excess gradient, as discussed earlier, is opposite to that expected for a diffusion-limited process. This observation, along with the negligible change in the electrostatic potential gradient near the surface established earlier ( Fig. 3b inset), is inconsistent with polaron migration between the bulk and the surface as rate determining. Further supporting this result is the excellent agreement between the polaron concentrations measured in this work and that measured under equilibrium conditions (zero current), also plotted in Fig. 4c . As in the case of oxygen vacancies, the variation in the surface polaron concentration with overpotential does not reflect slow kinetics. Rather, it reflects the quasi-equilibrium between bulk and surface polarons. Although the remarkable segregation of polaron at the surface reaction conditions mimics that of oxygen vacancies, its effect on the kinetics of the electrochemical incorporation reaction is expected to be substantially more pronounced because no polarons forms upon extrinsic aliovalent doping, and that the bulk Ce 3+ concentration can be as low as 9 × 10 −6 (relative to all Ce) at an overpotential of 0.35 V. Such an observation suggests that the abundance of Ce 3+ (surface electron) as another origin of the rapid incorporation kinetics, especially at HOR conditions under which the concentration of bulk electrons is negligible. Having obtained a holistic picture of the rapid reaction of hydroxyl with surface oxygen vacancies as well as the facile bulk-to-surface transport of both oxygen vacancies and small polarons (summarized in Fig. 5a ), we now turn our attention towards identifying the likely rate-determining step. The steady-state nature of our in operando measurement prevents the rates of elementary steps involving short-lived intermediate species from being assessed directly. Instead of expressing the reaction pathway as a collection of true elementary steps, we present a simplified electrochemical pathway, which proceeds via the intermediate based on our observations ( Fig. 5b ). The division of the reaction steps is arbitrary to some extent and does not necessarily indicate the stability of the minority intermediate species. Shown schematically in the WSR direction, step (1) and (2) are the H 2 O adsorption and dissociation steps, respectively. It is followed by electron transfer (3), hydrogen association (4) and H 2 desorption (5). Finally, the surface is regenerated to the initial state via bulk-to-surface mass transport (6). Given the moderate deviation from equilibrium, we assume the reaction pathway in the forward direction is identical to that in the reverse direction. 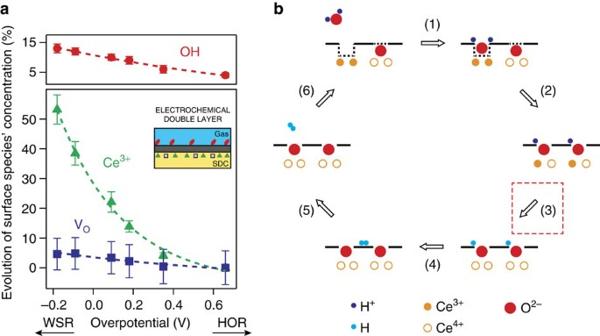Figure 5: Speculating the reaction pathway at the SDC–gas interface. (a) Dynamics of surface reactive species in the ceria–gas electrochemical interface. The dashed lines are for guiding the eyes. Oxygen vacancy concentration was determined usingSupplementary Equation 2based on the relative change in the total O 1s photoemission intensity. The error bars account for the uncertainties from the normalization and peak fitting process. (b) Schematic diagram of the proposed reaction pathway in the WSR direction. Simplified significantly to illustrate essential features of the reaction pathway. The reaction begins with H2O adsorption (1) and dissociation (2), and is followed byreduction (3), H association (4) and H2desorption (5). Finally, the system returns to the initial state through mass transport of small polarons and oxygen ions from the bulk to the surface (6).reduction (3) is the likely rate-determining step. Figure 5: Speculating the reaction pathway at the SDC–gas interface. ( a ) Dynamics of surface reactive species in the ceria–gas electrochemical interface. The dashed lines are for guiding the eyes. Oxygen vacancy concentration was determined using Supplementary Equation 2 based on the relative change in the total O 1s photoemission intensity. The error bars account for the uncertainties from the normalization and peak fitting process. ( b ) Schematic diagram of the proposed reaction pathway in the WSR direction. Simplified significantly to illustrate essential features of the reaction pathway. The reaction begins with H 2 O adsorption (1) and dissociation (2), and is followed by reduction (3), H association (4) and H 2 desorption (5). Finally, the system returns to the initial state through mass transport of small polarons and oxygen ions from the bulk to the surface (6). reduction (3) is the likely rate-determining step. Full size image Our observation that the surface oxygen vacancy is fully saturated with hydroxyl ions under both WSR and HOR conditions unambiguously rules out steps (1) and (2) as rate determining. Likewise, bulk-to-surface transport of both oxygen vacancies and polarons (6) is not rate determining, as evidenced by the negligible transport overpotential. By a process of elimination, our analysis leaves the electron transfer (step (3)), hydrogen association/dissociation (step (4)) and H 2 desorption/adsorption (step (5)) as potentially rate determining during WSR and HOR. The decrease in the surface hydroxyl concentration with anodic polarization is consistent with step (4) as rate determining. However, based on the current-voltage characteristics ( Supplementary Fig. 6 ), the absence of a current-limited behaviour on both the anodic and cathodic branches suggests that the rate-determining step cannot be a non-electrochemical step that occurs before or after all electron and ion charge-transfer steps, namely steps (1), (4) and (5) [2] , [26] . In other words, non-zero charge-transfer coefficient for both WSR and HOR suggests that the non-electrochemical adsorption or desorption is not likely the rate-determining step. Combined, the above evidence leads us to speculate that the small polaron transfer (step (3)) from Ce to surface hydroxyl group in WSR is most likely rate determining: where the species resides on surface oxygen vacancies. Sometimes, steps (3) to (5) are considered as a single step, namely H 2 desorption/adsorption with charge transfer. Our proposal is also consistent with such a combined step as rate determining. We note that the above rate-determining step differs from that recently proposed by Zhang et al. [32] , which employed an argument based on the accumulation and depletion of surface species. As shown in this work, such an argument does not readily apply to oxygen-incorporation oxides where the concentrations of bulk oxygen vacancy and mobile electron depend strongly on the overpotential, and the surface and bulk species are coupled via quasi-equilibrium segregation. We also acknowledge that reaction barriers might change with Ce 3+ and vacancy concentration and could complicate the above analysis. For example, increasing adsorbate concentration upon cathodic bias could lead to adsorbate–adsorbate interaction, which has been predicted in the case of CO 2 adsorption [56] . Such an interaction could in turn drive the non-electrochemical reactions, even though only neutral species are involved. The plausible rate-determining step proposed above suggests avenues for improving the electro-catalytic activity of ceria and other oxygen-ion incorporation materials. Because the surface is nearly saturated with and localized electrons, lowering the formation energy of these species is not expected to affect the reaction rate constant significantly. Instead, efforts should focus on lowering the barrier height for the electron transfer between Ce 3+ and , namely, decreasing the misalignment of the Ce 4f electronic state and the valence electrons in the adsorbate. Such an insight may also apply to other oxygen-incorporation solids with surfaces saturated with oxygen vacancies. In summary, direct spectroscopic quantification of the ceria–gas interface revealed the surface oxygen-ion incorporation pathway during electrochemical hydrogen oxidation and water splitting. We observed the facile reactivity of oxygen vacancies with water molecules, sustained enrichment of both oxygen vacancy and small polaron defects on the surface, and the rapid rates at which additional vacancies and polarons are transported between the bulk and the surface. These in operando observations suggest that electron-transfer step, rather than the ion-transfer step, is rate-determining during incorporation. We propose that the fast ion transfer is responsible for the facile surface incorporation activity of doped cerium oxide under WSR and HOR, and potentially of other oxides as well. By understanding the roles of surface oxygen vacancies and electrons in determining the rate of incorporation reactions, this work provides the fundamental insight necessary to optimize the activity of oxide electrodes rationally. Sample preparation The model electrochemical cells were fabricated on 10 × 10 × 0.5 mm 3 (100) Y 0.16 Zr 0.84 O 1.92 (YSZ) single-crystal substrates (one side polished, MTI Corporation), which serve as the oxygen-ion-conducting solid electrolyte. The fabrication procedure is described below in chronological order. First, the counter electrode was fabricated. A thin-layer Sm 0.2 Ce 0.8 O 1.9 (SDC) of about 50 nm was grown on the rough side of YSZ substrate by pulsed-laser deposition (PLD). The target fabrication procedure was reported previously [17] . Deposition was performed at a temperature set point of 750 °C in 0.5 mTorr O 2 using Coherent LPX-200 KrF 248 nm excimer laser (1 J cm −2 , 4 Hz). Serving as the co-catalyst, porous Pt thin film (~80 nm thick) was then deposited on top of the SDC by d.c. magnetron sputtering in 75 mTorr of Ar. The high activity and large area of the counter electrode guaranteed the counter-electrode reaction did not limit the cell. This is evident in the precise matching between the core-level binding energy shifts and the overpotential ( Fig. 3b ). Next, the Pt patterned current collector was fabricated on the smooth side of the substrate using metal lift-off photolithography ( Supplementary Fig. 7 ). Positive photoresist (Shipley S-1813) was spin-coated onto the polished side of YSZ substrate at 4,000 r.p.m. for 45 s and baked at 115 °C for 150 s. After aligning the mask with the substrate using a Karl Suss MJB 3 mask aligner, the sample was exposed to ultraviolet light for 17 s. Then the photoresist was developed in Microposit Developer solution for 50 s. After rinsing with deionized water and drying, the developed pattern was further cleaned by oxygen plasma etching. Metallization was then performed in the same sputtering system, where 170 nm Pt was deposited in 9 mTorr Ar. Metal lift-off followed by immersing the sample in acetone at room temperature. The fabricated patterns were 12 × 1,820 μm stripes separated by 6 μm spacing. The total 15 stripes were interconnected at the ends by a 500 × 500 μm 2 Pt contact pad. This dimension was optimized for efficient electronic conduction while maintaining good ionic conduction. Before the final deposition of the SDC thin film, the top and bottom Pt films were annealed at 600 °C in 860 Torr H 2 /H 2 O (8:1) atmosphere for 3 h. Finally, a 450-nm thick SDC thin film was deposited by PLD. An Inconel shadow mask with an opening of 0.5 × 2 mm was employed to deposit SDC on top of the Pt patterned current collector. The PLD deposition was performed at 700 °C in 5 mTorr O 2 with laser fluency 0.5 J cm −2 at 10 Hz. Electrochemical XPS APXPS were performed at beamline 9.3.2, Advanced Light Source, Lawrence Berkeley National Laboratory. The beamline is equipped with a differentially pumped Scienta R4000 HiPP electron analyser, which allowed the sample to be exposed to a gas atmosphere up to 1 Torr (ref. 28 ). Our homebuilt sample holder provides both heating and electrical contacts [57] . The sample was mounted onto the heater with a wound Pt wire sandwiched in-between for electrical connection with the bottom (counter) electrode. Au/Pd-coated W probes contacted the top (working) electrode. The catalytic effect from the low surface area probe (placed ~1 mm from the XPS analysis area) is expected to be small, as recently shown by Chueh et al. [17] During the experiment, the sample was first heated in 4.5 × 10 −5 Torr of O 2 to remove the adventitious carbon on the sample surface. Then 260 mTorr H 2 /H 2 O/Ar mixture (8:1:4) was introduced to provide the reaction environment. After the polarization experiment, the chamber was pumped out to high vacuum (10 −7 Torr) to check residual adsorbates on sample surface. In H 2 /H 2 O/Ar mixture, different voltage biases were applied between the top and bottom electrodes using a Bio-Logic SP-300 potentiostat. The temperature was monitored by measuring impedance of the YSZ substrate. The dependence of the YSZ impedance on temperature was calibrated in an ex-situ tube furnace. Soft X-ray shined onto the sample surface at an incident angle of 75° with respect to sample normal. At each polarization, core-level and valence band spectra were collected at an acceptance angle parallel to sample normal. Various photon energies were used to attain different information depths. For surface-sensitive measurements, the kinetic energies of the photoelectrons were controlled at approximately 160–250 eV; for more bulk-sensitive measurements, kinetic energy of ~680 eV was used ( Supplementary Table 1 ). The top electrode and a piece of Au foil on the sample surface were Fermi coupled with the electron analyser. The binding energy of each spectrum was calibrated using Au 4f 7/2 peak. How to cite this article: Feng, Z. A. et al. Fast vacancy-mediated oxygen ion incorporation across the ceria–gas electrochemical interface. Nat. Commun. 5:4374 doi: 10.1038/ncomms5374 (2014).